Dual-channel spontaneous emission of quantum dots in magnetic metamaterials Metamaterials, artificial electromagnetic media realized by subwavelength nano-structuring, have become a paradigm for engineering electromagnetic space, allowing for independent control of both electric and magnetic responses of the material. Whereas most metamaterials studied so far are limited to passive structures, the need for active metamaterials is rapidly growing. However, the fundamental question on how the energy of emitters is distributed between both (electric and magnetic) interaction channels of the metamaterial still remains open. Here we study simultaneous spontaneous emission of quantum dots into both of these channels and define the control parameters for tailoring the quantum-dot coupling to metamaterials. By superimposing two orthogonal modes of equal strength at the wavelength of quantum-dot photoluminescence, we demonstrate a sharp difference in their interaction with the magnetic and electric metamaterial modes. Our observations reveal the importance of mode engineering for spontaneous emission control in metamaterials, paving a way towards loss-compensated metamaterials and metamaterial nanolasers. The control of spontaneous emission in photonic structures relies on enhanced light–matter interactions because of field localization and large interaction times [1] , [2] , [3] . As such, nanostructured plasmonic materials are well suited for this purpose because they offer strong field confinement and can be engineered to support good coupling to free space, thereby opening up a way towards applications such as quantum information devices [4] , [5] , solar-energy harvesting [6] , efficient photodetection [7] , [8] and biological markers [9] . At the same time, the opportunity of reducing losses and achieving gain in plasmonic structures using quantum emitters is particularly promising for optical metamaterials, in which the step to practical applications is significantly hindered by energy dissipation in metals. Overcoming this major obstacle would lead to novel functional materials based on the control of both electric and magnetic material responses at optical frequencies, namely, to negative refractive index [10] , [11] , [12] , chirality [13] , [14] , [15] , [16] , [17] , [18] and subwavelength imaging [19] as well as to compact nanolasers and spasers [20] , [21] . Finally, active metamaterials might also enter new, unexplored areas such as quantum metamaterials [22] , [23] , [24] . In recent years, strong efforts have been made to find practical ways of reducing losses in optical metamaterials [21] , [25] , [26] , [27] , [28] , [29] , leading to the first demonstration of a loss-compensated negative-index metamaterial [26] . An important step in controlling the process of loss compensation is the study of coupling of quantum emitters such as quantum dots (QDs) with metamaterials. In such structures, the hybridization of QDs with electric resonances of a metamaterial can lead to photoluminescence (PL) enhancement and modification of the PL properties that can be controlled by the metamaterial design [30] , [31] . Topological transitions in hyperbolic metamaterials [32] have also shown an important avenue to alter the photonic density of states by changing the isofrequency surfaces via plasmonic resonances. However, when there are two modes involved, such as electric and magnetic modes in negative-index metamaterials, these modes provide different routes for the extraction of energy from the emitters. As such, an important question is how the energy of the emitter is distributed between these two modes and whether any of these modes dominates the emission dynamics. To date, an analysis of the PL emission properties for different metamaterial modes and specifically the control of emission via electric and magnetic modes have not been reported. Here we study experimentally the emission enhancement in a system of QDs coupled to a magnetic metamaterial consisting of split-ring resonators (SRRs), the prototype magnetic metamaterial [33] , [34] , [35] , [36] characterized by several well-known plasmonic resonances [37] , [38] , [39] . In contrast to previous work investigating PL enhancement in single nanoparticles and nanoantennas [3] , [40] , [41] or in Fano-type [30] , [42] , [43] and hyperbolic metamaterials [31] , [32] , our SRR metamaterial supports both electric and magnetic modes that are spectrally matched to the emission of semiconductor QDs at around λ QD =800 nm wavelength. Since both modes in our metamaterial can be engineered independently from each other, our QD metamaterial offers new opportunities to tailor the spontaneous emission of quantum emitters into two independent radiative decay channels. We demonstrate that the emission of QD metamaterials is fundamentally different for the magnetic and electric modes of the SRR metamaterial, revealing the interplay between the Purcell enhancement and energy coupling to free space. Remarkably, we observe that the magnetic mode, characterized by strong contributions of non-radiating higher multipole moments, exhibits stronger PL enhancement than the dipole-like electric mode. This is unlike the case of small, highly symmetric metal particles in which PL enhancement is governed by the dipole moment of the nanoparticle [40] , [44] while higher-order excitations cannot couple to the far field and lead to PL-quenching. Furthermore, in sharp contrast to the previous work on coupling of metamaterials to semiconductor quantum wells [27] , coupling of QDs to different plasmonic modes is not restricted by selection rules imposed by the quantum-well structure. Hence, core-shell QDs are a highly flexible and robust material system that allow for investigating mode competition in QD-metamaterial systems. Metamaterial mode analysis The system investigated here consists of a SRR metamaterial covered by a 200-nm-thick layer of polyvinyl alcohol (PVA) containing a low concentration of core-shell colloidal QDs emitting around λ QD =800 nm wavelength (for details see Methods). The sample geometry is depicted in Fig. 1 . The SRR metamaterial is designed in such a way that both its magnetic and electric modes are superimposed with the emission of semiconductor QDs. 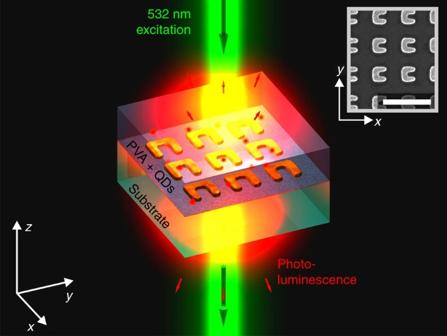Figure 1: Sample geometry. Artist’s impression of the sample geometry (not to scale): A magnetic SRR metamaterial processed on a glass substrate is covered by a 200-nm-thin PVA layer containing QDs. The sample is excited by 532-nm cw laser from the top with a × 100 objective (NA=0.9). The measured spot size was ~800 nm. The QD PL is then collected from the bottom. The inset shows a scanning electron micrograph of a sample without the QD-containing PVA layer. The scale bar is 500 nm. Figure 1: Sample geometry. Artist’s impression of the sample geometry (not to scale): A magnetic SRR metamaterial processed on a glass substrate is covered by a 200-nm-thin PVA layer containing QDs. The sample is excited by 532-nm cw laser from the top with a × 100 objective ( NA =0.9). The measured spot size was ~800 nm. The QD PL is then collected from the bottom. The inset shows a scanning electron micrograph of a sample without the QD-containing PVA layer. The scale bar is 500 nm. Full size image Linear-optical transmittance spectra of the metamaterial samples after spin-coating of the QD layer have been collected using a white-light spectroscopy setup and an optical spectrum analyser. Three different sets of split-ring-resonator metamaterials, marked as samples A, B and C, have been characterized for x - and y polarization of the incident light. These results are depicted in Fig. 2a,b also including a typical measured QD-PL spectrum of uncoupled QDs (PL 0 ) visualizing the sample- and the mode-dependent spectral overlap of the QD-PL spectrum with the plasmonic modes of the split-ring-resonator metamaterial. In both polarizations, the characteristic (higher-order) plasmonic resonances [37] , [38] , [39] are clearly visible in the spectral region of interest between 700 and 1,000 nm wavelength. 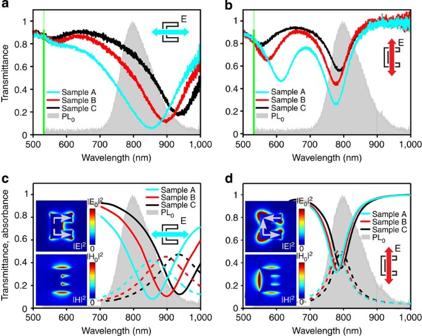Figure 2: Linear-optical properties of the quantum-dot metamaterial. (a,b) Measured transmittance spectra for the SRR metamaterial covered by the QD-PVA layer for the incident electric-field polarized inx- andydirections, respectively. Different curves correspond to samples with slightly different parameters. The grey-shaded region shows a typical measured free-space QD-PL spectrum PL0; the vertical green line indicates the excitation wavelength for PL measurements. (c,d) Calculated transmittance (solid lines) and absorbance (dashed lines) spectra (without QDs). The insets show calculated electric and magnetic field intensities of the corresponding modes for sample A, both normalized to the same maximum intensity (and, respectively). The electric dipole moments in each individual arm of the SRR are schematically indicated as grey arrows. Figure 2: Linear-optical properties of the quantum-dot metamaterial. ( a , b ) Measured transmittance spectra for the SRR metamaterial covered by the QD-PVA layer for the incident electric-field polarized in x - and y directions, respectively. Different curves correspond to samples with slightly different parameters. The grey-shaded region shows a typical measured free-space QD-PL spectrum PL 0 ; the vertical green line indicates the excitation wavelength for PL measurements. ( c , d ) Calculated transmittance (solid lines) and absorbance (dashed lines) spectra (without QDs). The insets show calculated electric and magnetic field intensities of the corresponding modes for sample A, both normalized to the same maximum intensity ( and , respectively). The electric dipole moments in each individual arm of the SRR are schematically indicated as grey arrows. Full size image In accordance with previous work [39] , [45] , [46] , the resonance excited in x polarization is characterized by a strong electric dipole moment [39] , which is naturally accompanied by strong radiative losses and, hence, a broad spectral line width; we therefore refer to this mode as the electric mode. In contrast, the resonance that is excited in y polarization is characterized by a superposition of an electric dipole, an electric quadrupole and a weaker magnetic dipole moment [39] and results in a narrower spectral linewidth of the resonance as compared with the electric mode. Owing to the presence of magnetic (multipole) moments, we refer to this mode as the magnetic mode (the fundamental magnetic mode of the SRR metamaterial is at 1.5 μm wavelength). From the transmittance spectra in Fig. 2a,b , we can extract the linewidths for the two modes at the resonance frequency . Owing to the different radiative properties of the electric and magnetic modes, this results in different linewidths, namely , 76 THz (B) and 65 THz (C) for the electric mode, as compared with , 39 THz (B) and 38 THz (C) for the magnetic mode. This is reflected in different quality factors for the two modes and allows us to identify the strongly radiating electric mode as the brighter mode and the magnetic mode, with its non-radiating quadrupole moment as the darker mode of the SRR metamaterial. In order to map our measurements to a simple model, we numerically calculate the transmittance spectra for the three samples (see Methods). These results are shown in Fig. 2c,d . Our calculations furthermore give us additional information about the optical near-fields and the electric moments of the two plasmonic modes. Normalized electric and magnetic field-intensity cross-sections calculated for the experimental parameters of sample A in the x–y plane cutting through the SRR are shown in the insets. The dipole moments in each individual arm of the SRR depicted in Fig. 2c,d also clearly visualize the quadrupole contributions to the magnetic resonance ( Fig. 2d ), while the electric resonance ( Fig. 2c ) is dominated by a strong electric dipole contribution. Furthermore, we calculate the effective mode volume V m of the two SRR modes and the fraction η of QDs located in the mode volume, hence, coupled to the metamaterial by evaluating the mode-volume integral [47] , [48] of a single SRR (see Methods). Since the mode volume is symmetric around the SRR at z =0 and extends approximately halfway into the PVA layer (with QDs), this gives us a fraction of QDs inside the mode volume. PL properties Next, the coupled QD-metamaterial system is investigated with respect to the luminescence properties for the electric and magnetic SRR modes. The QDs are excited off-resonantly at λ =532 nm to investigate the emission processes in the coupled QD metamaterial at around λ =790 nm. Note that the excitation wavelength is well below the SRR resonances (see Fig. 2a,b ), where the transmittance of the metamaterial is close to unity. Hence, we can assume that the presence of the metamaterial is not significantly affecting the excitation rate of the QDs. Using an analyser in the detection path allows us to independently select the x - and y -polarized QD-PL components of the randomly positioned and oriented QDs. In the following, we discuss the experimental results of spatial QD-PL mapping ( Fig. 3a,b ) and spectrally resolved QD-PL measurements ( Fig. 3c,d ) for sample A. This sample has the strongest spectral overlap of the QD luminescence with both metamaterial modes and, therefore, the strongest coupling efficiency. Additionally, the transmittance for the two different linear polarizations, corresponding to the two plasmonic modes, takes on approximately the same value of about 28% at λ =790 nm close to the central wavelength λ QD of the QD-PL emission. 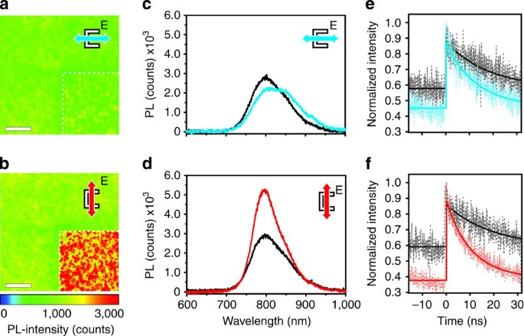Figure 3: PL properties of the coupled QD-metamaterial system. (a,b) Confocal mapping of the QD PL is shown forx-polarized andy-polarized detection, respectively. The metamaterial is situated in the lower right corner of the images, as indicated by the white-dashed lines. The scale bars are 6 μm. (c,d) Measured QD-PL spectra forx- andypolarization are plotted in blue and red, respectively. The reference QD PL (PL0) is shown in black. (e,f) Measured time-resolved QD PL (dashed lines) normalized to its maximum value and fitted exponential decays (solid lines) forx- andypolarization plotted in blue and red, respectively. Figure 3: PL properties of the coupled QD-metamaterial system. ( a , b ) Confocal mapping of the QD PL is shown for x -polarized and y -polarized detection, respectively. The metamaterial is situated in the lower right corner of the images, as indicated by the white-dashed lines. The scale bars are 6 μm. ( c , d ) Measured QD-PL spectra for x - and y polarization are plotted in blue and red, respectively. The reference QD PL (PL 0 ) is shown in black. ( e , f ) Measured time-resolved QD PL (dashed lines) normalized to its maximum value and fitted exponential decays (solid lines) for x - and y polarization plotted in blue and red, respectively. Full size image Figure 3a,b shows the spatially mapped QD PL both on the metamaterial sample (lower right corner of each image) and next to the metamaterial for x and y orientations of the polarizer in the detection path, respectively. The QD-PL maps in Fig. 3a,b show that for y -polarized detection (magnetic mode) the PL-enhancement factors are on average ~1.5; however, there are spatial positions where enhancement of up to approximately three can be observed. This is a notable enhancement given that, in contrast to single plasmonic structures [3] , [40] , [49] where a precise placement of the emitters is possible [40] , [41] , [50] , large PL-enhancement factors are harder to realize in metamaterials since, here, the main focus is on the spatially averaged effective response of the coupled QD metamaterial. For this reason, in our experiments and numerical simulations, we average over all possible distances, lateral positions and dipole orientations of the QDs with regard to the split-ring-resonator meta-atom. In this way, we perform statistical averaging in order to adequately compare the coupling of the QDs to both modes of the split-ring-resonator metamaterial and obtain an averaged enhancement factor of ~1.5 in the experiment. In contrast to the magnetic mode, for the electric mode ( x -polarized detection) the effective magnitude of the PL intensity is not significantly changed by the presence of the metamaterial. Hence, for the electric mode the PL enhancement and the losses of the coupled system are balanced, resulting in an averaged PL-enhancement factor close to unity. Since the fraction of QDs near the metal surface is low, quenching of the QD emission cannot be held responsible for the low PL-enhancement factor of only the electric mode. On the contrary, the changes in the shape of the PL spectrum shown in Fig. 3c are a clear indication that the QDs are indeed coupled to the electric mode of the SRR metamaterial. Line-shape distortions are also observed for the magnetic mode of the coupled system and demonstrate the coupling of the QDs to the two different modes in the SRR metamaterial. Remarkably, in our experiment the magnetic mode, which exhibits weaker coupling to the far-field, as evidenced by narrower and less pronounced resonances in transmittance measurements ( Fig. 2b,d ), and which can thus be considered as the darker mode, becomes the brighter mode in the QD emission ( Fig. 3b,d ). These results are further supported by micro-PL spectra that depict the influence of the metamaterial on the spectral shape of the QD emission. In these measurements, we have collected QD-PL spectra at selected bright spots on the SRR metamaterial and from the reference area. A typical experimental micro-PL spectrum for sample A for x -polarized and y -polarized QD emission is shown in Fig. 3c,d , respectively. Consistent with our results from spatial PL mapping, we observe PL enhancement and a narrowing of the QD-PL spectrum for y -polarized emission, while for x -polarized emission broadening of the QD-PL spectrum is observed. We note that, while the maximum measured PL intensity varies for different spots on the metamaterial sample because of slightly different distances of the QDs to the plasmonic structures in the metamaterial, the overall spectral shape of the emission is maintained for different spots. To investigate the overall performance of the QD metamaterial in terms of PL enhancement, we additionally show histograms of the PL-intensity distribution ( Fig. 4 ) extracted from the spatial mapping data shown in Fig. 3a,b , confirming an average measured PL enhancement of ~1.66 for the magnetic mode of sample A. 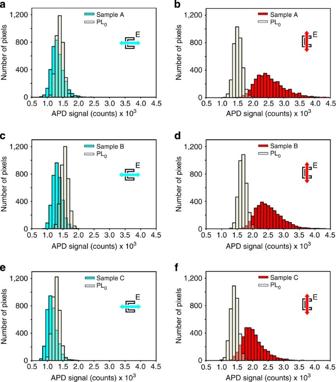Figure 4: PL-intensity statistics. (a,b) PL histograms for sample A showing the spatial PL-intensity distribution of the QD emission on the metamaterial and on the reference area (PL0) extracted fromFig. 3a,bfor (a)xpolarization and (b)ypolarization. (c–f) show the corresponding data for samples B and C, respectively. Figure 4: PL-intensity statistics. ( a , b ) PL histograms for sample A showing the spatial PL-intensity distribution of the QD emission on the metamaterial and on the reference area (PL 0 ) extracted from Fig. 3a,b for ( a ) x polarization and ( b ) y polarization. ( c – f ) show the corresponding data for samples B and C, respectively. Full size image In order to further support our results, we perform time-resolved PL measurements for samples A–C around λ =780 nm wavelength and compare them with the corresponding measurements on reference areas without metamaterial. The lifetime measurements for sample A are depicted in Fig. 3e,f . The PL-decay times for the two modes are extracted by fitting exponential functions to the experimental data. While the decay curves obtained for the reference areas look very similar for x - and y polarizations ( and ), we measure a clear decrease in PL lifetime for the QDs coupled to both the electric ( ) and the magnetic modes ( ) of sample A and observe that the decrease is more pronounced for the magnetic mode in y polarization. For samples B and C, we obtain for the electric mode—that is, slightly increasing lifetimes—in contrast to slightly decreasing lifetimes for the magnetic mode when comparing samples A–C. Hence, for all three samples we find a distinct difference in lifetime between the two modes, providing clear evidence that the previously observed PL enhancement is indeed an effect of the QDs coupling to the modes of the metamaterial. Toy model of the coupled system In order to understand the non-trivial connection between the measured PL enhancement and the Purcell factor, we develop a simple toy model of the PL enhancement and decay times and compare these estimates with our experimental findings. In our toy model, we account for plasmonic field confinement, off-resonant coupling and scattering properties of the different metamaterial resonances. While this model does not fully describe the complex QD–plasmon interaction and neglects the influence of uncontrolled parameters because of sample imperfections, variations in gold quality (surface roughness), and shape variations of the QDs, it can nevertheless be used to understand the mechanisms that govern the QD-PL modification in presence of the metamaterial. In our approach (see also Methods), assuming saturation of QD excitation, we can estimate the measured PL-enhancement factor Y where η is the fraction of QDs that is actually contained inside the mode volume V m and is coupled to the near-field of the SRRs. T is the experimental transmittance value for the corresponding mode of the metamaterial sample at the emission wavelength of the QDs, and F p,mod is the Purcell factor of our combined system: The total density of states of the plasmonic cavity mode and the spectral distribution of optical transitions in the (homogeneously broadened) emitter are both described by normalized Lorentzian functions with resonance frequencies and linewidths . The plasmonic resonances coupled to the QDs are described by the parameters and extracted from the experimental transmittance spectra of the SRR modes. We also note that in contrast to the uncoupled fraction of QDs, the coupled system of QDs and metamaterial is characterized by the modified radiative and non-radiative losses, hence a (modified) quantum yield. Using the central QD-emission wavelength λ QD =800 nm, the effective refractive index of the SRR environment n =1.45, and the transmittance/linewidth for the x - and y -polarized modes from the transmittance spectra ( Fig. 2a,b ), we calculate the enhancement factors , for the electric mode, and , for the magnetic mode, respectively. These results are in good agreement with the experimental values and they correspond to the calculated Purcell factors , 1.66(B), 1.34(C) and , 3.06(B), 3.23(C) of the QDs which are coupled to the metamaterial modes only. For better quantitative comparison with the experimental PL-mapping data, Fig. 4a,b shows histograms of the intensity distribution of the QD emission obtained from the spatial PL data shown in Fig. 3a,b . The corresponding experimental data for samples B and C are shown in Fig. 4c–f , respectively. Extracting the median values for the PL intensity of the QD reference and the PL of the QD metamaterial, we can calculate the median experimental PL enhancement for samples A–C. For the electric mode, we obtain enhancement factors , while for the magnetic mode significantly higher values are measured. The PL enhancement of the two modes is also in good agreement with numerical PL-enhancement calculations using CST Microwave Studio (see Methods). As a next step, we estimate the upper limit for the lifetimes of the coupled QD metamaterials using (see Methods): ( q being the quantum yield of the QDs) and compare them with the experimental data. We obtain values of for the electric mode and for the magnetic mode. Being upper-limit estimates for the lifetimes, they agree well with the experimentally measured values. In particular, the main experimental observation that the decay into the magnetic mode happens faster than into the electric mode is very well reproduced by our simple model. Furthermore, the predicted trends that the lifetimes are getting shorter/longer from sample A to sample C for the magnetic/electric mode can also be found in the experiment. However, because of the occurrence of additional non-radiative decay channels in the experiment, there are deviations of the toy-model prediction from the experimental values for the PL lifetimes and for the PL-enhancement factors. These additional non-radiative losses can mainly be attributed to fabrication imperfections (gold quality, gold-surface roughness) of the different SRR-metamaterial samples, which cannot be fully captured by the ideal parameter set used to describe the QD-PL properties and the plasmonic cavity. Hence, when comparing the PL measurements of samples A–C we observe that the PL enhancement for the magnetic mode is gradually reduced, while a slight increase is predicted by our simple model. Furthermore, while the qualitative trends of the PL lifetimes are reproduced by the toy model, there are small deviations in the absolute numbers in experiment and in the toy model. Both effects can be linked to an increase in non-radiative losses in the experiment that may be very different for the different samples. As the third observation, we can compare the spectral line shape of QD PL for coupling to the two different modes and for a varying spectral overlap of the QD PL and the metamaterials’ resonances (samples A–C). 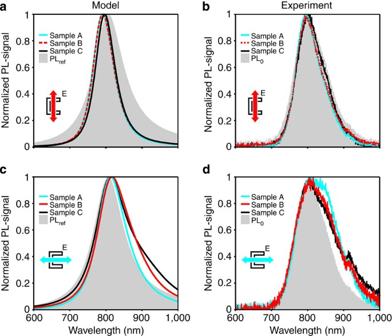Figure 5: Line-shape distortion. Predicted and measured normalized micro-PL spectra for the magnetic (a,b) and electric (c,d) modes for samples A, B and C plotted in blue, red and black, respectively. The measured PL of the uncoupled QD emission (PL0) and the modelled reference QD-PL shape (PLref) are indicated as grey-shaded area. While for coupling to the electric mode (c,d) broadening and distortion of the PL emission are predicted and observed, the PL for coupling to the magnetic mode (a,b) shows a narrowing with regard to the reference QD PL. Figure 5 shows spectrally resolved PL for ( Fig. 5a,b ) magnetic and ( Fig. 5c,d ) electric modes on normalized scale to allow for easy comparison of the line shapes with the reference QD-PL also shown in Fig. 5 . In contrast to the case of a single emitter at low temperatures, where the spectral width is determined by the total decay rate, in our experiment the spectral overlap of the (broadened) QD PL with the electric and magnetic modes of the SRRs results in a distortion of the PL spectra. In the experiment ( Fig. 5b,d ), we observe a broadening for x -polarized detection (electric mode) in ( Fig. 5d ) and a narrowing for y -polarized detection (magnetic mode) in ( Fig. 5b ) for all samples. Moreover, shape variations can clearly be identified among the three different samples, particularly for the electric mode, where the spectral mode position for sample A to sample C gradually shifts out of resonance with the QD PL. In order to compare these experimental findings with predictions from our simple model, we calculate the PL line shape along the lines of Tanaka et al. [30] Generally, the PL line shape consists of an enhanced and spectrally modified contribution from the coupled QDs, and an undisturbed contribution from the uncoupled QDs, yielding Figure 5: Line-shape distortion. Predicted and measured normalized micro-PL spectra for the magnetic ( a , b ) and electric ( c , d ) modes for samples A, B and C plotted in blue, red and black, respectively. The measured PL of the uncoupled QD emission (PL 0 ) and the modelled reference QD-PL shape (PL ref ) are indicated as grey-shaded area. While for coupling to the electric mode ( c , d ) broadening and distortion of the PL emission are predicted and observed, the PL for coupling to the magnetic mode ( a , b ) shows a narrowing with regard to the reference QD PL. Full size image These results are given in Fig. 5a,c , and they reproduce well the experimental trends. In particular, the broadening for the electric and narrowing for the magnetic modes and the change of line shape for the electric mode are nicely reproduced. Summarizing our experimental findings, we have demonstrated, for the first time to our knowledge, the coupling of QDs to a magnetic split-ring-resonator metamaterial at near-infrared frequencies. Via polarization-dependent spatially-, spectrally-, and time-resolved QD-PL measurements, we have demonstrated that the PL enhancement, spectral shape and lifetime of the QD-metamaterial emission are strongly dependent on the SRR-mode properties involved in the process. By deliberately designing the SRR metamaterial to support electric and magnetic modes overlapping with the QD emission, we are able to investigate coupling of QDs to two different radiative channels at the same time. We observe PL enhancement of the QD emission of up to a factor of 3 with respect to the QD emission without metamaterial for emission into the magnetic mode, which is characterized by additional electric quadrupole and magnetic dipole moments. PL enhancement into the electric channel, on the other hand, is close to unity. At the same time, the QD lifetime in the coupled QD metamaterial is shortened by a factor of ~2. We also find that in contrast to small spherical metal particles, the contribution of higher-order electric moments to the radiative emission properties is substantially increased and even leads to greater PL enhancement factors for the magnetic mode than for the electric dipole mode. This finding also has important implications for the design of plasmonic nanostructures for emission enhancement—for example, in single-molecule and fluorescence-sensing applications [50] . As opposed to small spherical nanoparticles in which higher-order modes are completely dark and can even cause PL-quenching, more complex structure designs make higher-order plasmonic modes accessible for PL enhancement, resulting in a more efficient detection of quantum emitters or molecules. In our experiment, we have collected data for three different metamaterial samples (see Supplementary Table S1 ) to investigate the influence of spectral overlap and resonance strength on the PL spectra of the QD metamaterial. Figure 5 demonstrates that the emission properties are also dependent on the spectral overlap of the QD PL and resonance position of the metamaterial mode. Our experiments are supported by calculations from our simple toy model in which the metamaterial modes are treated as optical microcavities coupled to a dipole emitter. The expected values for PL enhancement, PL lifetimes and PL line shape of the QD-metamaterial emission are in good agreement with the experimental values for the two SRR-metamaterial modes. Our novel approach of using plasmonic mode engineering to tailor spontaneous emission of QD metamaterial systems provides an important insight to the enduring problem of loss compensation in metamaterials by gain media. In particular, when the electric and magnetic modes of a metamaterial are overlapping (such as in negative-index metamaterials), there will be competition for the extraction of the accumulated energy in the emitter. This affects the effective permittivity and permeability and, hence, the effective impedance of the metamaterial. This change of the impedance under the presence of gain is known as gain-induced impedance mismatch in the metamaterial, as recently predicted theoretically [51] . The gain-compensation efficiency can then be controlled by engineering of the overlapping modes and, hence, by precise adjustment of the metamaterial parameters. Furthermore, we believe that our findings show a significant impact on new concepts of metamaterials, such as the control of emission of quantum light from quantum emitters coupled to the metamaterial. An interesting example could be engineering the emission of entangled photon pairs from bi-excitonic excitations in QDs, which are emitted in two orthogonal polarizations [52] , [53] . According to our findings, one of the possible two-photon decay channels would be favoured by the presence of the SRR metamaterial, allowing for tailoring the probabilities of the two orthogonal states to occur. Sample preparation The split-ring-resonator metamaterials (design parameters: lattice constant a =300 nm, x -width l x =131 nm, y -width l y =148 nm, widths of the two arms w x =48 nm, width of the central arm w y =69 nm) have been fabricated via standard electron-beam lithography on a glass substrate covered by a 5-nm indium-tin-oxide layer, subsequent evaporation of 20±2 nm of gold and a lift-off procedure. A scanning electron microscopy image of a typical sample is depicted in the inset of Fig. 1 . The dimensions for the SRRs are extracted from the scanning electron microscopy images and varied within the tolerances of extraction so that the numerical spectra match the experimental ones. The lateral SRR dimensions of samples B/C are taken as , , the widths of the two arms are and the width of the central arms are . After fabrication of the metamaterial samples, a 50:50 mixture of PVA solution (60 gl −1 PVA 98–99% hydrolysed, Sigma Aldrich, in H 2 O) and a core-shell QD solution (CdSeTe core with a shell of ZnS and polymer coating in 10 μl, 2.2 μM Invitrogen Qdot800 ITK streptavidin conjugate, quantum yield q =56% (lot data), diluted in 500 μl Invitrogen Qdot800 incubation buffer) have been processed on top of the metamaterial sample by spin-coating (3,000 r.p.m., 90 s). PVA has previously been shown to form a viable transparent matrix for CdSe–ZnS QDs, leading to stable QD luminescence and no quenching effects being observed [54] . The resulting PVA–QD layer thickness has been measured to be using a Tencor alpha-step 200. The calculated density of the QDs in the PVA is ~0.2 QDs per metamaterial unit cell, which has to be considered as a lower bound taking into account the shrinkage of the PVA layer upon drying. This low concentration of QDs was chosen to provide a homogeneous distribution of QDs in the PVA and prevent clustering. The system of CdSeTe/ZnS/polymer QDs in PVA is chosen because of its high photobleaching threshold, good thermostability, chemical resistance, easy processability and transparency in the relevant spectral region. Numerical calculations For calculating the transmittance spectra and field distributions of the SRR-metamaterial samples, we use the finite-element frequency-domain solver of the software package CST Microwave Studio with adaptive mesh size. The lateral dimensions of the SRRs (sample A) are taken as , , the widths of the two arms is and the width of the central arm is . To avoid sharp edges that could give rise to numerical artefacts, we introduce round edges with a curve radius of 2 nm. The SRRs are arranged in a periodic lattice with the lattice constant a =300 nm. The gold thickness is 20 nm. For modelling the gold, we use a Drude model with a plasma frequency of and a damping of . These values were obtained by fitting the Drude formula to the experimental values for the permittivity of gold in the visible/near-infrared spectral region [55] with a slightly increased damping to match the experimental depth and width of the SRR resonances. The refractive indices of the glass substrate is taken as , of the 5-nm-thin indium-tin oxide layer as , and for the PVA layer we take . Numerical calculation of the mode volume In order to calculate the effective mode volume for the magnetic and electric modes at the centre wavelength of the QD emission, we numerically calculate the electric fields of a single SRR with the dimensions of sample A. The SRR is embedded in a homogeneous medium ( ) so that the resonance positions of the SRR are located at the same spectral position as for the periodic case (see Fig. 2 ). Since the height of the (planar) SRR is only 20 nm, the incident field for the calculation of the mode volume is strictly identical along the extent of the SRRs (for normal incidence) and we can apply the quasi-static approximation [56] to calculate the mode-volume integral for a leaky plasmonic cavity [47] , [48] This equation is a widely used measure for the mode volume of plasmonic cavities in the literature [57] , [58] , [59] . Here is the average energy density experienced by a randomly positioned emitter in the simulation volume (which is, truncated at the boundaries of the metamaterial unit cell and the height of the QD-containing PVA layer (see inset in Fig. 6 ). For the calculation of the energy density in the homogeneous medium, we use and for the metal we use [47] , where γ is the Drude damping of gold. The permittivity of gold is taken from our simulations. Finally, we calculate the extent of the mode volume in the z direction (light-shaded area in the inset in Fig. 6 ) by dividing Equation 5 by the unit-cell area and obtain the total z height of the mode volume (indicated in Fig. 6 ) after subtraction of the linear divergence (dashed lines in Fig. 6 ). Since the mode volume extends symmetrically from to , we conclude that the mode volume extends approximately halfway into the QD-containing PVA layer. This also gives us the fraction of QDs inside the mode volume , where is the volume of the PVA layer with the thickness h in a unit cell with the lattice constant a . 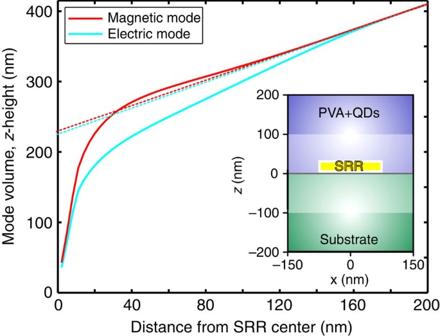Figure 6: Mode-volume calculation. Mode volume integral for the magnetic (red) and electric (blue) modes of a single SRR embedded in an effective medium, evaluated atλQD=800 nm and plotted over thezdistance to the SRR centre. The dashed lines represent the linear divergence due to radiation loss for the two modes. The intersection of the dashed lines with theyaxis at aroundzm=226 nm defines the totalzheight of the mode volume (light-shaded area) for a unit cell area of 300 nm × 300 nm. Figure 6: Mode-volume calculation. Mode volume integral for the magnetic (red) and electric (blue) modes of a single SRR embedded in an effective medium, evaluated at λ QD =800 nm and plotted over the z distance to the SRR centre. The dashed lines represent the linear divergence due to radiation loss for the two modes. The intersection of the dashed lines with the y axis at around z m =226 nm defines the total z height of the mode volume (light-shaded area) for a unit cell area of 300 nm × 300 nm. Full size image PL-mapping and PL-spectroscopy setup Micro-PL spectroscopy and micro-PL spatial mapping have been performed using a commercial WITec alpha300S system in confocal microscope configuration (for further details see Supplementary Fig. S1 ). In this setup, a 532-nm continuous-wave laser is focused on the sample with a × 100 objective ( NA =0.9) from the PVA side for excitation of the QDs. The measured spot size was ~800 nm. The QD PL is then collected from the substrate side of the sample using a × 50 ( NA =0.65) infrared-corrected objective (transillumination mode). A linear polarizer inserted into the detection path allows for selectively collecting the PL for x - and y polarization. In order to remove the light of the exciting laser source from the signal, a Semrock NF 03-532E-25.4-D notch filter has been introduced. The spectrometer is fibre-coupled to the microscope using a multimode (non-polarization maintaining) fibre to neutralize any possible polarization sensitivity of the gratings. To further rule out any unwanted effects from the excitation source, we have used the same excitation scenario for all measurements and we checked that the polarization of the exciting laser has no significant influence on the behaviour of the detected QD-PL. We chose an average excitation power below the destruction threshold of the SRR metamaterial while, at the same time, maximizing the signal-to-noise ratio. In this excitation regime, the QD-PL signal increases sublinearly with excitation power, indicating that we are pumping the QDs well beyond the onset of the saturation regime [60] . Owing to the damage threshold of the gold SRRs, however, we do not quite reach the ideal saturation regime; hence, an increase in excitation power is still connected to a slight increase in PL signal. For spatial mapping, the QDs have been excited with an average power of ~0.34 mW, leading to an excitation power density of ~80 kWcm −2 on the sample. The PL has been collected for x - and y polarization using an avalanche photodiode in combination with a band-pass filter. For micro-PL spectroscopy, the QDs are excited with approximately twice the power density than for the spatial mapping in order to obtain a sufficiently high signal. For detection of the PL spectra, we have used a Princeton Instruments ACTON SP 2300 spectrometer connected to an InGaAs spectroscopy CCD detector (Andor Technology DU491A-1.7-352) and a low-pass filter with 630-nm cutoff wavelength in order to filter out any remaining parasitic radiation. An integration time of 100 s has been used, which is required because of the low efficiency of the InGaAs detector at these frequencies, as well as because of the coupling losses into the fibre connectors. Time-resolved PL setup Time-resolved measurements of the QD-metamaterial PL at λ =780 nm wavelength were carried out at room temperature in air. In this setup (see Supplementary Fig. S2 ), a 522-nm solid-state pulsed laser (20.8 MHz) was focused at an average power of 24.5 μW through a × 50 objective lens ( NA =0.55) on the sample with a beam waist of around 2 μm. The emitted PL was detected in reflection mode using a single-photon avalanche photodiode and a time-correlated single-photon counting system with an instrument response of ~50 ps at full-width-at-half-maximum, resulting in an integration time of 10 s. In addition, a linear polarizer was used in the detection path to discriminate between the PL emissions of the two modes. The lifetimes of the QDs in the reference area have been obtained by fitting a single exponential function to the experimental data. For fitting of the PL intensity I p from the metamaterial region, we use a double-exponential function with weight factors for the two decay channels proportional to the fraction of the detected light emitted by the QDs coupled ( ηF p,mod ) and not coupled [(1- η )(1+ R )] to the metamaterial. Here R is the reflection of the metamaterial at 780 nm wavelength, accounting for the reflection geometry used in experiment. The decay time of the uncoupled QDs is fixed to the decay time of the reference QD PL . For the two modes in the two polarizations, this yields This modelling accounts for the contribution of the coupled QDs in the lower part of the PVA as well as for the contribution of the uncoupled QDs positioned in the upper half of the PVA layer and the reflection of the metamaterial. We note that, in contrast to the PL-mapping system, the excitation power and integration times are significantly lower at comparable signal counts. Toy-model description of the system In our simple toy model we treat each mode of the SRR metamaterial equivalent to a microcavity with resonance frequency ω cav , linewidth and an ultrasmall (open) mode volume V m [30] , [61] , [62] . The maximum Purcell factor for optimal spatial and polarization overlap is then given by [61] , [62] where n is the refractive index of the medium and is the emitter wavelength. The total density of states of the plasmonic cavity mode can be described by a normalized Lorentzian function centered at ω cav with a linewidth of Δ ω cav We note that by assuming a Lorentzian function for the linewidth of the QD emission, we neglect shape variations of the QDs themselves that lead to an inhomogeneous line broadening in the experiment. Nevertheless, our toy model takes off-resonant coupling into account, which is particularly important for samples B and C. Since, additionally, the cavity linewidth and the linewidth of the QDs are comparable, , in the above expression has to be replaced by the spectral overlap integral where is a normalized Lorentzian function describing the spectral distribution of optical transitions in a homogeneously broadened emitter [61] . Despite some inhomogeneous broadening of the QD PL in the experiment caused by averaging over a small ensemble of QDs in our experiment, we still approximate as a Lorentzian function in our simple model, obtained by fitting a Lorentzian line shape to the measured QD PL spectrum. This results in the modified Purcell factor If the system is pumped in the saturation regime of excitation, the luminescent level of the QDs is always populated and the intensity enhancement factor F PL = τ r,QD / τ cav,r is independent of the quantum yield q . Here τ cav,r is the radiative lifetime of the coupled system and τ r,QD is the radiative lifetime of the free QDs. Assuming an ideal cavity dominated by strong radiative losses, F PL can be approximated by the Purcell factor F p,mod = τ r,QD / τ cav , where τ cav is the total lifetime of the coupled system. To finally obtain the observable quantity, namely the PL intensity, from F PL , we furthermore have to account for the fraction of QDs that are actually contained inside the mode volume (light-shaded area in Fig. 6 ), where is the part of the plasmonic mode volume overlapping with the PVA volume within a unit cell ( ). Since the QD PL is detected in transillumination mode, we approximate the PL signal from the uncoupled QDs that is transmitted through the sample by multiplying the original emission from the uncoupled QDs with the transmittance T of the metamaterial mode. This leads to a measured PL-enhancement factor Y of Note that the measured enhancement for the coupled QDs, namely the first term of the above expression, is independent of the mode volume. The second term accounts for the PL contribution to the measured signal caused by the uncoupled QDs in the upper half of the PVA layer. Given the Purcell factor, we can calculate the lifetime of the QD-metamaterial system via [63] where is the non-radiate lifetime of the QDs in the coupled system. Assuming that the non-radiative lifetime of the QDs in the coupled QD-metamaterial system is equal or smaller than the QD’s free-space non-radiative lifetime , we can use the QD’s measured free-space total radiative lifetime and their quantum efficiency . We can then determine the lifetime of the coupled QD metamaterials via , and which finally results in Following Tanaka et al. [30] , we can also estimate the line shape of the measured PL by taking both the PL contribution of the QDs coupled to the metamaterial (first term) and the transmitted PL contribution of the uncoupled QDs (second term) into account. The results of the toy-model calculations are summarized in Supplementary Table S1 . Naturally, deviations arise from the fact that the toy model does not take all experimental details into account. For instance, the toy model cannot fully map the variations with regard to losses/non-radiative decay within the SRRs arising from variations of gold quality because of different degrees of surface roughness for the samples A–C. Particularly, when approaching the fabrication limit by reducing the linewidth of the gold SRRs, the losses between the different samples may change significantly. However, a detailed analysis of this aspect is far from trivial and beyond the scope of our work. Additionally, the orientation of the QDs with respect to the electric-field components is important when calculating the PL-enhancement factor. Since this aspect is not accounted for in our toy model, this results in an overestimation of the PL enhancement. Another factor contributing to overestimation of the PL enhancement by our toy model, which, however, does not affect the lifetime estimates, is the assumption of an ideal cavity dominated by strong radiative losses. Finally, we neglect deviations originating from directional emission of QDs in combination with the limited collection angle in detection in the experiment. Although this effect might play a role, our tests using a dedicated back-focal plane setup indicate that deviations originating from directional emission are small. Generally, despite the limitations of our simple model, the quantitative values obtained from the toy model fit the experimental values well, hence, allowing us to make qualitative predictions about the effect of different mode overlaps and mode characteristics on the measured PL enhancement in our system. Numerical simulations of PL enhancement To further test the prediction of our toy model, we performed direct numerical simulations using CST Microwave Studio and the sample parameters for sample A. We simulate the emission of a point-dipole oriented in x -, y - and z directions, respectively, and subsequently detect the QD emission in x - and y direction of polarization. We performed calculations of PL spectra for a quantum emitter situated in a plane at distances of d =5, 25, 45, 65 and 85 nm above the split-ring-resonator metamaterial and for several (30) positions of the dipole within each plane (see inset in Fig. 7 ). We then average over the PL-enhancement values at each position and each distance d for x -polarized and y -polarized emissions. The PL-enhancement spectra for x - and y -polarized emissions of the dipoles are normalized to the emission of the reference point-dipole source. In doing so, we map the exponentially decaying electric fields of the SRR modes with a step width of 20 nm, keeping the simulation time at reasonable time scales. Furthermore, we avoid numerical artefacts because of the step-like change in permittivity from gold to the surrounding medium by starting the simulation at d =5 nm above the gold surface. The resulting numerical PL-enhancement spectra are depicted in Fig. 7 for the magnetic and electric modes ( y - and x -polarized emissions), respectively. For the spectral region around 790 nm (grey-shaded area), the numerical results confirm an average PL enhancement of 2.02 for the magnetic mode as compared with 1.67 for the electric mode. These values are larger than those in the experiment, since the resonance linewidths of the electric and magnetic resonances in the simulation are narrower than those in the experiment (see Fig. 2c,d ). As a result, the losses are smaller in the simulations and larger PL-enhancement factors are expected. Despite the larger losses in the experiment, we still observe a qualitatively good agreement between our numerical calculations and our experimental results. Particularly, since the PL enhancement for the magnetic mode is a factor of 1.21 larger than for the electric mode and the spectral distortion of the QD-PL is very well reproduced, our numerical calculations are consistent with the experiment and the results from the toy model. 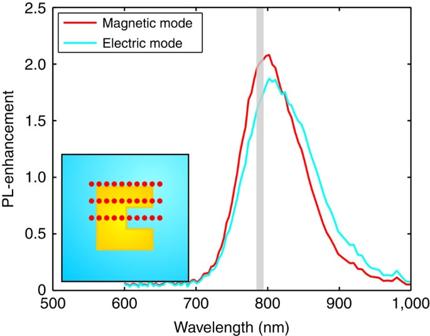Figure 7: Numerical PL enhancement spectra. PL-enhancement spectra for the magnetic (red) and electric (blue) modes of the SRR averaged over all spatial positions indicated by the red dots in the inset. The raw data are normalized to the emission of an undisturbed point dipole and multiplied with the normalized experimental PL spectrum of the QDs. Figure 7: Numerical PL enhancement spectra. PL-enhancement spectra for the magnetic (red) and electric (blue) modes of the SRR averaged over all spatial positions indicated by the red dots in the inset. The raw data are normalized to the emission of an undisturbed point dipole and multiplied with the normalized experimental PL spectrum of the QDs. Full size image How to cite this article: Decker, M. et al. Dual-channel spontaneous emission of quantum dots in magnetic metamaterials. Nat. Commun. 4:2949 doi: 10.1038/ncomms3949 (2013).